Efficient genome engineering by targeted homologous recombination in mouse embryos using transcription activator-like effector nucleases Generation of mouse models by introducing transgenes using homologous recombination is critical for understanding fundamental biology and pathology of human diseases. Here we investigate whether artificial transcription activator-like effector nucleases (TALENs)—powerful tools that induce DNA double-strand breaks at specific genomic locations—can be combined with a targeting vector to induce homologous recombination for the introduction of a transgene in embryonic stem cells and fertilized murine oocytes. We describe the generation of a conditional mouse model using TALENs, which introduce double-strand breaks at the genomic locus of the special AT-rich sequence-binding protein-1 in combination with a large 14.4 kb targeting template vector. We report successful germline transmission of this allele and demonstrate its recombination in primary cells in the presence of Cre-recombinase. These results suggest that TALEN-assisted induction of DNA double-strand breaks can facilitate homologous recombination of complex targeting constructs directly in oocytes. Current research in life sciences relies heavily on sophisticated genetic mouse models allowing cell- and tissue-specific expression or knockout of conditionally targeted alleles utilizing Cre-recombinase technology. A major bottleneck of current technology is the necessity to introduce transgenes by homologous recombination in ES cells, often a labour-intensive, error-prone and time-consuming process. Therefore, large consortia have been established to effectively address these issues [1] . Over the last 2 years, site-specific gene targeting to incorporate locus-specific DNA double-strand breaks using transcription activator-like effector nucleases (TALENs) has been introduced [2] , [3] . This technology has been successfully applied in several animal models including mouse, rat, zebrafish and Caenorhabditis elegans [4] , [5] , [6] , [7] , [8] . Gene targeting via non-homologous end-joining (NHEJ) has also been suggested to generate combined reporter and knockout alleles [9] . Combination of TALEN-based gene targeting with insertion of a few base pairs or transgenes using small ssDNA oligonucleotides or donor vectors with longer homologous arms was initially reported for zebrafish [10] , [11] and later extended to other animal models including mouse [12] , [13] . The mouse remains the most widely used animal model in the study of human biology and diseases. Since tissue-specific gene modification is highly desirable, we investigate whether this new technology can be translated to conditional targeting of a genomic allele of higher vertebrates such as the mouse using large targeting constructs. To our knowledge, a mouse line harbouring a conditionally targeted allele has not previously been created by combined injection of TALENs with a targeting construct into mouse embryos, allowing for homologous recombination at a specific site in the mouse genome. Here we induce a conditional allele at the gene locus of the special AT-rich sequence-binding protein-1 (Satb1), a factor known to recruit chromatin-remodelling enzymes that is required for normal thymic T-cell development [14] , TH1/TH2 polarization [15] , [16] , and reprogramming of gene expression [17] specifically suppressed in T reg cells [18] . This allele simultaneously combines loss of endogenous Satb1 expression with eGFP reporter activity under the endogenous regulatory elements normally driving SATB1 expression. The targeting vector is optimized for TALEN-based strategies and can be readily adapted to other genes within the mouse genome. In addition, we apply an improved methodology to screen for TALEN-mediated nuclease activity utilizing an in vitro approach based on an in vitro transcription and translation system [10] . Taken together, we show successful homologous recombination at the Satb1 locus directly in fertilized oocytes, thereby demonstrating that injection of TALEN mRNA together with complex targeting constructs into oocytes facilitates the generation of conditionally targeted animals. Generation of a targeting vector for the murine Satb1 locus To test whether homology-directed repair of a specific genomic locus is possible in vivo in mouse embryos, we generated a targeting construct for the murine Satb1 locus with 1.8 kb 5′ and 4.9 kb 3′ homology arms. This construct contained exon 2 comprising the start codon for Satb1 within a FLEX switch [19] , allowing for a Cre-recombinase mediated exchange of exon 2 with an artificial exon 2 encoding for the endogenous 5′ untranslated region (UTR) and the start codon fused to eGFP. Within the targeting construct, eGFP was directly followed by the 3′ UTR of Satb1 to enable the regulation of the reporter gene by endogenous miRNAs previously reported to fine-tune Satb1 expression ( Supplementary Fig. 1 ) [18] , [20] . Assessment of recombination efficacy revealed a 100% success rate in prokaryotes expressing Cre-recombinase ( Supplementary Fig. 2 ). eGFP expression was tested in the human embryonic kidney cell line 293 T and the murine fibroblast cell line NIH3T3. Co-transfection of a eukaryotic expression vector containing the FLEX switch together with a Cre-recombinase containing plasmid led to robust eGFP fluorescence ( Fig. 1a–c and Supplementary Fig. 3 ), while no fluorescence was detected following transfection of HEK293T cells with the FLEX construct alone ( Fig. 1a–c and Supplementary Fig. 3 ). These results suggested that the targeting construct was fully functional in vivo . 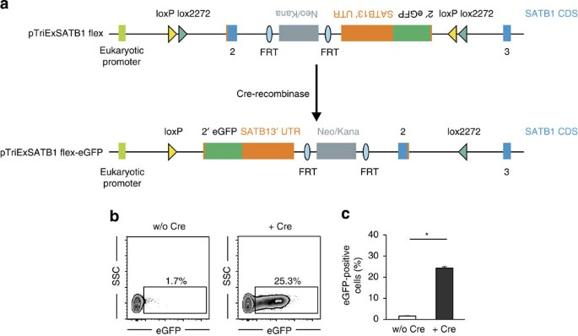Figure 1: Functionality of the eGFP-expressing modified FLEX switch within the conditional targeting construct for the murineSatb1locus. (a) Schematic of the FLEX switch contained in the conditional targeting construct for the murineSatb1locus transferred to an eukaryotic expression vector before and after Cre-recombinase induced recombination. (b,c)In vivorecombination of the FLEX switch in HEK293T cells 24 h after transfection. eGFP expression was determined by flow cytometry in control (w/o Cre) or Cre-recombinase co-transfected cells (+Cre). (b) Exemplary dot plots of a single experiment. (c) Quantification of eGFP expression (n=3). Mean and s.e.m. *P<0.05 (Student’st-test). Figure 1: Functionality of the eGFP-expressing modified FLEX switch within the conditional targeting construct for the murine Satb1 locus. ( a ) Schematic of the FLEX switch contained in the conditional targeting construct for the murine Satb1 locus transferred to an eukaryotic expression vector before and after Cre-recombinase induced recombination. ( b , c ) In vivo recombination of the FLEX switch in HEK293T cells 24 h after transfection. eGFP expression was determined by flow cytometry in control (w/o Cre) or Cre-recombinase co-transfected cells (+Cre). ( b ) Exemplary dot plots of a single experiment. ( c ) Quantification of eGFP expression ( n =3). Mean and s.e.m. * P <0.05 (Student’s t -test). Full size image Generation of a TALEN pair for the murine Satb1 locus To target the murine Satb1 locus we designed and synthesized highly active TALENs that bind to an intronic region of the murine Satb1 locus contained within the FLEX switch ( Fig. 2a ). We used an in vitro assay system based on in vitro transcription and translation of the TALENs to exclude TALEN pairs with low efficiencies in inducing DNA double-strand breaks before assessing their activity in vivo [10] . We showed TALEN protein activity against a PCR product of the targeted locus and demonstrated high rates of DNA double-strand break induction ( Fig. 2b ). We then used this TALEN pair for the classical T7 in vivo assay analysing TALEN activity in NIH3T3 cells ( Fig. 2c,d ). Taken together, these data demonstrate successful generation of a TALEN pair directed at a sequence just upstream of exon 2 inducing small deletions at its target site. 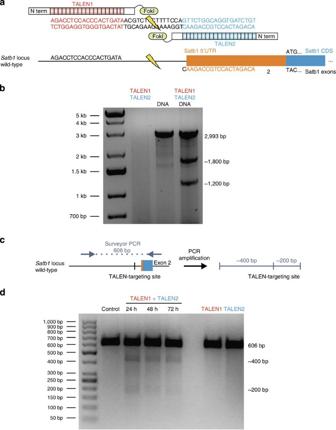Figure 2: Generation of TALENs targeting the murineSatb1locus. (a) Schematic showing the layout of theSatb1TALEN target site with DNA-binding sequences (in red or blue) and the spacer region of 15 bp. (b) In a cell-freein vitrotranscription and translation system generatedSatb1TALENs were active against a PCR product spanning the TALEN-targeting site at the genomicSatb1locus. (c) Schematic representation of the PCR reaction amplifying the TALEN-targeting region as well as the two products resulting from T7 endonuclease I-mediated fragmentation of DNA-heteroduplexes. (d) T7 endonuclease I assays were conducted using PCR-amplified genomic DNA from TALEN-transfected NIH3T3 fibroblasts (TALEN 1+TALEN 2) or control transfected cells to assessin vivoefficacy of theSatb1TALENs. Size of the PCR product as well as the size of T7 endonuclease I-digested DNA fragments is depicted on the right. Control, negative control. Figure 2: Generation of TALENs targeting the murine Satb1 locus. ( a ) Schematic showing the layout of the Satb1 TALEN target site with DNA-binding sequences (in red or blue) and the spacer region of 15 bp. ( b ) In a cell-free in vitro transcription and translation system generated Satb1 TALENs were active against a PCR product spanning the TALEN-targeting site at the genomic Satb1 locus. ( c ) Schematic representation of the PCR reaction amplifying the TALEN-targeting region as well as the two products resulting from T7 endonuclease I-mediated fragmentation of DNA-heteroduplexes. ( d ) T7 endonuclease I assays were conducted using PCR-amplified genomic DNA from TALEN-transfected NIH3T3 fibroblasts (TALEN 1+TALEN 2) or control transfected cells to assess in vivo efficacy of the Satb1 TALENs. Size of the PCR product as well as the size of T7 endonuclease I-digested DNA fragments is depicted on the right. Control, negative control. Full size image As this TALEN pair is directed against an intronic region at the Satb1 locus also contained in the targeting construct ( Supplementary Fig. 1 ), we modified the Satb1 -targeting construct to include three point mutations at the binding site of each TALEN to prevent TALEN-induced modification of the targeting construct and subsequently of the targeted Satb1 allele. TALEN-assisted homologous recombination in ES cells Recent in vivo work in zebrafish and mice has demonstrated that small stretches of homologous DNA as well as donor vectors with longer homologous arms can be used for homology-directed repair based genome editing at a TALEN-induced double-strand break. Thus, we hypothesized that the combined injection of the TALEN mRNA pair together with the modified 14.4 kb Satb1 targeting construct into the male nucleus of mouse pronuclear-stage embryos and subsequent transfer into foster mice could also result in successful homologous recombination of the Cre-recombinase dependent conditional genetic allele and produce homologously recombined or mutant founders (F0). Prior to oocyte injections, we tested the function of TALENs and TALEN-mediated homologous recombination in JM8A3 embryonic stem cells. Using standard methodology we were unable to obtain any correctly targeted ES cells from 56 surviving clones ( Table 1 ). In contrast, using a combined transfection of TALEN DNA and the targeting construct, 30.1% ( n =41) of the 136 surviving clones showed correct integration at the 5′ and 3′ end. Taken together, these results indicate that TALEN-mediated induction of DNA double-strand breaks favors homologous integration in ES cells and could be a valuable tool to improve targeting efficiency. Table 1 TALEN-mediated Satb1 gene targeting in JM8A3 ES cells. Full size table Generation of a conditional Satb1 mouse strain Based on our encouraging results, we injected TALEN mRNA and the targeting construct into oocytes from B6D2F1 × C57BL/6J mice. Injections of nearly 900 oocytes gave rise to 67 newborns, which were assessed for homology-directed repair and genomic modifications ( Table 2 ). Table 2 TALEN-mediated Satb1 gene targeting in B6D2F1 × C57Bl/6J mice. Full size table First, we determined efficacy of genomic modifications for two different concentrations of Satb1 TALEN mRNA (10 and 5 ng μl −1 ) using a combined endonuclease treatment and sequencing approach of the PCR-amplified TALEN-targeting site ( Supplementary Fig. 4 ). 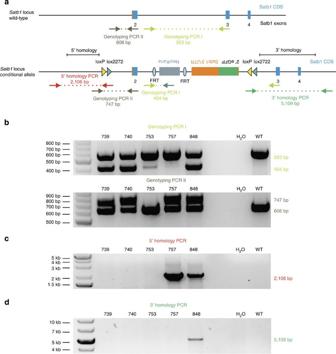Figure 3: Germline integration of the conditional targeting construct at the genomicSatb1locus. (a) Schematic of the murine wild-typeSatb1locus and the targetedSatb1allele with binding regions of the respective oligos for the PCR screening forin vivorecombination. Genotyping PCR I in lime green, oligo only binding on targeting construct in dark green; genotyping PCR II in grey, 5′ homology region spanning PCR (5′ homology PCR) in red; 3′ homology region spanning PCR (3′ homology PCR) in green. (b) Germline screening of theSatb1locus. Tail biopsies from 67 founders were pre-screened with the two genotyping PCRs and 5 founders showed at least one positive result in one of the genotyping PCRs. (c) These were assessed for recombination in the 5′ region with the 5′ homology region spanning PCR. Two mice demonstrated precise germline homology-directed repair in the 5′ region. (d) Analysis of 3′ integration by PCR. The mouse showing homologous recombination at the 5′ region also shows integrationviahomology-directed repair at the 3′ end. In line with recent findings, the majority of TALEN-induced mutations were deletions of variable length ( Table 3 ) yielding 17 mutants (25.4%) with 4 mutant mice carrying bi-allelic mutations. In one mouse two differently mutated alleles and the wild-type allele were detected, suggesting a TALEN-induced chimerism in this animal ( Table 3 ) [6] . TALEN activity appeared to be dose-dependent, since injections of the higher dose (10 ng μl −1 ) of Satb1 TALEN mRNA resulted in 5 of 11 (45.5%) F0 mice displaying TALEN-induced genomic modifications, while the lower concentration (5 ng μl −1 ) yielded 12 of 56 (21.4%) F0 mice carrying a mutation at the TALEN-targeting site ( Table 2 ). In contrast to recently published data on the generation of TALEN-induced knockout mice [6] , we did not observe a clear difference in the percentage of mutant mice produced per oocyte injected for both concentrations of TALEN mRNA (5/297, 1.7% versus 12/426, 2.8%). This result speaks against significant off-target effects as also supported by our off-target prediction ( Supplementary Table 1 ). Table 3 Sequencing of the TALEN-targeting site at the Satb1 locus in founder mice. Full size table Using a PCR-based screening approach ( Fig. 3a ), we assessed whether the Satb1 -targeting construct had integrated at any site in the genome. Among the 67 animals we identified 5 founder animals that were positive in at least one of these screens ( Fig. 3b , upper and lower panel). We then tested the five positive founder animals to see whether integration of the targeting construct had occurred via homology-directed repair in the 5′ homology region. This PCR analysis demonstrated somatic introduction of the Satb1 targeting construct at the genomic Satb1 locus on chromosome 17 in two founder animals ( Fig. 3c ). One of these animals was negative in the genotyping PCR I, which recognizes parts of the neomycin cassette, suggesting that homology-directed repair in this animal occurred via the targeted exon 2 contained within the FLEX switch. To determine whether integration in the 3′ homology region also occurred in the one founder animal positive in the genotyping PCRs and the 5′ homology PCR, we developed a long-range PCR to assess successful integration spanning the 4.9-kb 3′ homology region, and observed correct integration ( Fig. 3d ). Integration of the targeting construct in the genome of the two founders positive in the 5′ homology PCR was confirmed by mutation analysis of the Satb1 TALEN site by sequencing as we detected the modified TALEN-targeting site from the Satb1 targeting construct in both animals ( Table 3 ). In addition, by sequencing the Satb1 TALEN-targeting site, we identified a third animal with homology-directed repair. In this animal, sequences within short range of the TALEN-targeting site were used for homology-directed repair as only one TALEN-binding region showed the mutations introduced in the targeting construct while the other was negative for the mutations ( Table 3 ). This explained the negative results for this animal in the genotyping PCRs. Together, these results suggest that homology-directed repair occurred in 2 of the 5 founder animals showing a positive signal for the integration of parts of the targeting construct (40%) and that in 3 of the 17 founders with TALEN-induced genomic modifications homologous recombination was used as a repair mechanism (17.7%), while NHEJ occurred in the other animals ( n =14, 82.3%, Supplementary Fig. 4 ). Figure 3: Germline integration of the conditional targeting construct at the genomic Satb1 locus. ( a ) Schematic of the murine wild-type Satb1 locus and the targeted Satb1 allele with binding regions of the respective oligos for the PCR screening for in vivo recombination. Genotyping PCR I in lime green, oligo only binding on targeting construct in dark green; genotyping PCR II in grey, 5′ homology region spanning PCR (5′ homology PCR) in red; 3′ homology region spanning PCR (3′ homology PCR) in green. ( b ) Germline screening of the Satb1 locus. Tail biopsies from 67 founders were pre-screened with the two genotyping PCRs and 5 founders showed at least one positive result in one of the genotyping PCRs. ( c ) These were assessed for recombination in the 5′ region with the 5′ homology region spanning PCR. Two mice demonstrated precise germline homology-directed repair in the 5′ region. ( d ) Analysis of 3′ integration by PCR. The mouse showing homologous recombination at the 5′ region also shows integration via homology-directed repair at the 3′ end. Full size image Successful germline transmission of the targeted Satb1 allele To test whether the targeted allele could also be transmitted through the germline, we crossed the potential founder mouse to wild-type mice and examined the genotypes of F1 offspring via the PCR-based screening approach described above. Using this method we observed successful germline transmission of the targeted Satb1 allele ( Fig. 4a ). Consistent with the results for the founder mouse, we also observed correct 5′ and 3′ integration of the targeting construct ( Fig. 4b,c ), suggesting that its F1 progeny stably inherited the targeted Satb1 allele. Genomic integration of a single copy of the donor allele was also confirmed by Southern blotting ( Fig. 5a–d ). 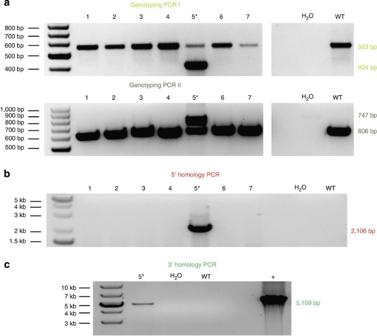Figure 4: Germline transmission of the conditional targeting construct at the genomicSatb1locus in F1 offspring. (a) Germline screening of theSatb1locus. Seven animals from the F1 generation were pre-screenedviatail biopsy. Of those pre-screened, one offspring (5*) was positive in both of the genotyping PCRs. (b) Analysis of 5′ integration by PCR. The one mouse positive in the screening PCRs (5*) shows germline transmission of the homologously recombined conditionalSatb1allele at the 5′ end. (c) Germline transmission of the conditionalSatb1allele to the F1 offspring was also confirmed by analysis of 3′ integration by PCR in animal 5*. Figure 4: Germline transmission of the conditional targeting construct at the genomic Satb1 locus in F1 offspring. ( a ) Germline screening of the Satb1 locus. Seven animals from the F1 generation were pre-screened via tail biopsy. Of those pre-screened, one offspring (5*) was positive in both of the genotyping PCRs. ( b ) Analysis of 5′ integration by PCR. The one mouse positive in the screening PCRs (5*) shows germline transmission of the homologously recombined conditional Satb1 allele at the 5′ end. ( c ) Germline transmission of the conditional Satb1 allele to the F1 offspring was also confirmed by analysis of 3′ integration by PCR in animal 5*. 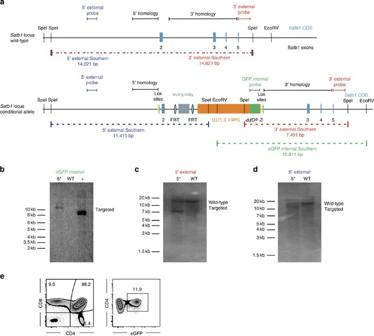Figure 5: Southern blot and functional assessment of the targetedSatb1locusin vivo. (a) Schematic of the murine wild-typeSatb1locus and the targetedSatb1allele with binding regions of the respective probes for Southern blot analysis. eGFP internal Southern blot in green; 5′ external Southern Blot in blue. 3′ external Southern Blot in red. (b–d) Southern blot analysis of single integration of the donor plasmidviahomologous recombination at the genomicSatb1locus using an eGFP internal (b), a 3′ external probe (c) and a 5′ external probe (d) on Eco RV (b) or Spe I (c,d) digested DNA. (e) Functionality of the targeted allele was assessed by flow cytometry in TAT-Cre-treated CD4+CD8+double-positive thymocytesin vitro. Full size image Figure 5: Southern blot and functional assessment of the targeted Satb1 locus in vivo . ( a ) Schematic of the murine wild-type Satb1 locus and the targeted Satb1 allele with binding regions of the respective probes for Southern blot analysis. eGFP internal Southern blot in green; 5′ external Southern Blot in blue. 3′ external Southern Blot in red. ( b – d ) Southern blot analysis of single integration of the donor plasmid via homologous recombination at the genomic Satb1 locus using an eGFP internal ( b ), a 3′ external probe ( c ) and a 5′ external probe ( d ) on Eco RV ( b ) or Spe I ( c , d ) digested DNA. ( e ) Functionality of the targeted allele was assessed by flow cytometry in TAT-Cre-treated CD4 + CD8 + double-positive thymocytes in vitro . Full size image Functionality of the FLEX switch in vivo To assess whether the targeted allele can be reversed by Cre-recombinase, we isolated thymocytes and splenocytes from the F1 progeny with one targeted Satb 1 allele and treated the cells in vitro with TAT-Cre recombinase. We found induction of eGFP expression after 24 h in double-positive thymocytes, indicating successful recombination of the targeted locus with subsequent expression of the reporter protein ( Fig. 5e ). In line with this observation, we also detected successful recombination in B cells and CD4 + and CD8 + T cells isolated from the spleen of these mice ( Supplementary Fig. 5a–c ), as well as in all relevant thymocyte populations ( Supplementary Fig. 5d–g ). Based on our promising in vitro results for ES cells demonstrating successful high-efficiency targeting of a locus previously shown to be relatively hard to target using classical targeting approaches, we hypothesized that co-injection of the targeting construct together with TALEN mRNA in murine oocytes could also be used to directly generate targeted mice carrying reporter and conditional alleles. To our knowledge, these results show for the first time in rodents that TALENs can be used to generate DNA double-strand breaks, which are subsequently repaired via homologous recombination using a large and complex co-injected targeting construct. Such an approach allows for the generation of a genetically targeted conditional allele in live embryos and ultimately in animals. Homology-directed repair in combination with TALEN-mediated genome editing has initially been described for zebrafish, where either short sequences (for example, loxP sites) were used as ssDNA donor templates for homology-directed repair [10] or donor vectors containing longer homologous arms up to 1 kb (ref. 11 ). While this manuscript was in preparation such findings have been extended to the mouse using a similar strategy for homologous recombination in mice that utilizes either short ssDNA donor templates or donor vectors to correct a single base mutation [12] , [13] . This work demonstrated that a donor vector with long homology regions, similar to the one used for this study, can be used for homology-directed repair in oocytes to exchange single base mutations. Our work now extends this finding to the integration of complex conditional alleles. Furthermore, more recent findings from the Jaenisch group have elegantly demonstrated that the CRISPR/Cas9 system can be used for genome engineering of mice [21] , [22] . In these elegant studies the CRISPR/Cas9 system was used to introduce DNA double-strand breaks in oocytes and co-injection of either short ssDNA or targeting plasmids resulted in homology-directed repair and correct recombination of the targeted allele in vivo [21] , [22] . Using two single-guide RNAs (sgRNAs) that target two regions flanking an exonic sequence even a conditional allele could be generated by providing short ssDNA encoding for loxP sites [22] . However, recombination with a complex conditional targeting plasmid or germline transmission of the targeted allele, as shown here, has not been reported to date for CRISPR/Cas9. It will be of great interest to perform studies comparing TALEN- versus CRISPR/Cas9- or ZFN-based approaches when engineering conditional alleles to identify advantages and disadvantages of these systems. Homologous recombination of the conditional Satb1 -targeting construct—which in total spans >14.4 kb and targets a region of 880 bp—suggests that genome engineering using TALENs in combination with homology-directed repair is not limited to the insertion of small oligonucleotides to generate conditionally targeted alleles. Instead it also allows for the complex engineering of a targeted locus using combined conditional knock-in–knockout alleles as demonstrated for the Satb1 FLEX construct. This is particularly remarkable as experiments in murine ES cells showed that our approach using this relatively large and complex targeting construct (for example, encompassing the 3′ UTR of Satb1) has only low rates of homologous integration, even under selection with G418 without TALEN-mediated induction of DNA double-strand breaks. In contrast, the rate of correctly recombined clones was increased if both TALENs and the targeting construct were transfected together. From these observations we conclude that the construct integration rate in oocytes, and the resulting frequency of homologously mutated animals, although slightly lower than reported (for example, for the ROSA26 locus using zinc-finger nucleases), is still within an acceptable range given the size of the targeting construct [23] , [24] , [25] , [26] . We observed TALEN-mediated induction of NHEJ in 25.4% of the offspring independent of targeting construct integration. These results are in line with efficiencies reported for zinc-finger nucleases in mice [25] , [26] , [27] and rats [28] , as well as for TALEN-injections in murine oocytes [6] , [12] , [13] , [29] . Newly established methodology using the CRISPR/Cas9 system to induce DNA double-strand breaks and facilitate homologous recombination [21] , [22] certainly raises high expectations that this system could also be used to mediate homologous recombination of larger donor plasmids directly in oocytes [22] . Initially, a potential danger of off-target effects was reported for the CRISPR/Cas9 system [30] , [31] , [32] , [33] . However, this limitation was recently overcome by introduction of a Cas9-based nickase in combination with two guide RNAs for homologous recombination [34] . Factors that could influence integration efficiencies after injecting a targeting plasmid together with TALEN mRNA directly into oocytes may include the targeting strategy itself (for example, the choice of the targeted exon), the size of the targeted gene, the size and complexity of the targeting plasmid, the length of the homology arms, the efficiency of TALENs to induce DNA double-strand breaks and the position of the TALEN-induced DNA double-strand break relative to the homology arms [35] . Future work should be directed towards comparative studies using different genome engineering technologies to understand whether certain loci might be more accessible for one but not another genome-editing technology. Certainly, for successful application of TALENs rigorous in vitro and in vivo testing of TALENs before injection into embryos is mandatory. To this end, we have adopted an efficient and fast in vitro approach to expedite the testing of TALEN pairs. An additional advantage of TALEN-mediated genome engineering is that once established, a TALEN pair (for example, for the ROSA26 locus), could be used to create multiple targeted mouse lines using different targeting constructs within a very short time frame. Using mice as model systems, we report somatic gene targeting with precise introduction of exogenous DNA sequences at one specific locus in embryos using TALEN-mediated genome editing combined with homology-directed repair resulting in the generation of a single transgenic founder animal. For zinc-finger nucleases, genome engineering using homology-directed repair has been well documented in murine oocytes using classical targeting approaches even for longer constructs and using homology arms as short as 800 bp (refs 23 , 24 , 25 , 26 ). However, considering the technological advantages provided by TALENs and the CRISPR/Cas9 system, an approach based on either of these newly established technologies is highly desirable. In general, by expediting and economizing TALEN and targeting vector generation, the described approach can be readily adapted to any other gene in the mouse genome and modified to integrate alternative reporter genes or read-out strategies. Furthermore, it will significantly accelerate the generation of highly sophisticated genetic mouse models. The introduction of the CRISPR/Cas9 system raises the question, which technology can be adopted for use on a larger scale to induce DNA double-strand breaks in oocytes. However, it is highly likely that every approach will have its specific application and that TALEN and CRISPR/Cas9 systems will be further developed in parallel. Taken together, genome engineering using the newly established TALEN and CRISPR/Cas9 systems could revolutionize somatic gene targeting as it bypasses the laborious, time-consuming and error-prone generation of targeted embryonic stem cells. We believe that both these technologies can potentially be applied to other animal models of higher vertebrates as well as many other species for which genetic engineering tools are needed. TALEN design and assembly TALENs targeting the murine Satb1 locus were designed using the TAL Effector Nucleotide Targeter [36] and assembled with the TALE toolbox following the published recommendations [37] . The plasmids for TALEN assembly were obtained from Addgene. Off-target prediction was performed using the TAL Effector Nucleotide Targeter 2.0 and the top potential off-targets are listed in Supplementary Table 1 . Amino acid sequences of the repeat variable di-residues of the Satb1 targeting TALENs are listed in Supplementary Table 2 . Cell culture and reporter activation assay Human embryonic kidney 293T (HEK293T) cells as well as NIH3T3 murine fibroblasts (both from ATCC) were maintained at 37 °C, 5% CO 2 , using Dulbecco’s modified Eagle’s Medium supplemented with 10% FBS, 2 mM GlutaMAX (Life Technologies), 100 U ml −1 penicillin and 100 μg ml −1 streptomycin. In vivo reporter assay for TALEN-mediated NHEJ In vivo activity of the murine Satb1 targeting TALEN pair was tested by transfecting NIH3T3 cells with plasmids encoding for the respective TALEN. NIH3T3 cells were seeded into six-well plates the day before transfection at densities of 2 × 10 5 cells per well. Approximately 24 h after initial seeding, cells were transfected using Turbofect (Fermentas). For six-well plates we used 4 μg of each TALEN plasmid per well. All transfection experiments were performed according to the manufacturer’s recommended protocol. After 24 to 48 h cells were harvested, DNA was isolated, and a region of 606 bp containing the Satb1 TALEN-targeting site was amplified by PCR and used for the T7 endonuclease I assays. To generate non-mutated DNA for the T7 endonuclease I assay, genomic DNA from NIH3T3 cells mock transfected with an eGFP plasmid was extracted and amplified by PCR. To allow complementary but mismatched strands to anneal, PCR products were mixed in NEB buffer 2 (10 × ) and incubated at 95 °C for 5 min, 95 °C to 85 °C at −2 °C s −1 and 85 °C to 25 °C at −0.1 °C s −1 . T7 endonuclease I (1 μl) (NEB) was added and samples were incubated at 37 °C for 60 min to digest the annealed PCR products at the sites of mismatch. T7 endonuclease I-digested PCR products were analysed by agarose gel electrophoresis. Oligonucleotide sequences used for PCR amplification of the DNA used for the T7 endonuclease I assay are listed in Supplementary Table 3 . In vitro assessment of TALEN-mediated genome editing To test for Satb1 TALEN activity in vitro we used the TnT Quick Coupled Transcription/Translation System (Promega) according to the manufacturer’s recommendations to transcribe and translate the TALEN encoding plasmids into TALEN proteins. After generation of TALEN proteins, a purified DNA fragment of 3.0 kb length containing the Satb1 TALEN-targeting site amplified from genomic DNA from NIH3T3 cells mock transfected with an eGFP plasmid was added to the reaction. After Proteinase K treatment and subsequent nucleic acid purification, TALEN activity was monitored by agarose gel electrophoresis. Oligonucleotide sequences used for PCR amplification of the DNA used for the in vitro test of TALEN activity are listed in Supplementary Table 4 . Microinjection into mouse embryos Mice were housed under specific pathogen-free conditions at the HET, University Hospital Bonn and used in accordance with the German legislation governing animal studies following ‘The Principles of Laboratory Animal Care’ (NIH publication no. 85-23, revised in 1996). Protocols for injections were reviewed and approved by the Animal Care Commission of North Rhine Westfalia, Germany (permit number: 8.87-50.10.31.09.042). Satb1 TALEN mRNAs were prepared using the mMESSAGE mMACHINE T7 Ultra kit (Ambion) according to the manufacturer’s instructions and diluted to working concentrations in diethyl pyrocarbonate (DEPC, Sigma)-treated injection buffer (0.25 mM EDTA, 10 mM Tris, pH 7.4). Two different concentrations (10 and 5 ng μl −1 ) of Satb1 TALEN mRNAs were injected together with 5 ng μl −1 of the targeting construct for the Satb1 locus into the male pronucleus of single-cell mouse embryos (B6D2F1 × C57BL/6J) in M2 medium (Sigma) using a Piezo-driven micromanipulator. After incubation at 37 °C for 4 h, non-lytic embryos were selected and transferred into the oviducts of pseudopregnant foster mothers. Genotyping of founder mice DNA was isolated from tail biopsies of the 67 (4 weeks of age, 36 ♀, 31 ♂) F0 founder mice (B6D2F1 × C57BL/6J) as well as 7 (4 weeks of age, 3 ♀, 4 ♂) F1 founder mice and germline transmission of the Satb1 targeting construct was evaluated using two screening PCRs: Satb1 genotyping PCR I using GoTaq DNA Polymerase (Promega) and Satb1 genotyping PCR II using Phusion Hot Start II Polymerase (Finnzymes). Homologous recombination at the Satb1 locus was assessed by PCR reactions using GoTaq DNA Polymerase with one primer located outside of the 5′ or 3′ homology region and the other only binding to the conditionally-targeted Satb1 allele but not to the wild-type Satb1 allele. PCR products were analysed by agarose gel electrophoresis. Oligonucleotide sequences used for PCR amplification of the DNA used for the genotyping are listed in Supplementary Table 5 . Analysis of founder mice for genome editing DNA was isolated from tail biopsies of founder mice, a region of 606 bp containing the Satb1 TALEN-targeting site amplified by PCR using Phusion Hot Start II Polymerase (Finnzymes) and used for the SURVEYOR nuclease assays. Briefly, the genomic region encompassing the TALEN target site was melted and re-annealed to form heteroduplex DNA. Nuclease S (0.5 μl) and Enhancer S (0.5 μl) (Surveyor Mutation Detection Kit, Transgenomic) were added and samples were incubated at 42 °C for 20 min to digest the annealed PCR products at the sites of mismatch. Nuclease S-digested PCR products were analysed by agarose gel electrophoresis. Oligonucleotide sequences used for PCR amplification are listed in Supplementary Table 3 . Sequence analysis of founder mice To confirm the genotype of F0 mice detected by SURVEYOR assays, PCR products were cloned into the pCRII-TOPO vector using the TOPO TA Cloning Dual Promoter Kit (Invitrogen) and mutations were identified by direct sequencing. Oligonucleotide sequences used for PCR amplification are listed in Supplementary Table 3 . Generation of the Satb1 targeting construct The Satb1 targeting construct was generated on the basis of the previously described FLEX switch obtained from Addgene [19] . First, the 5′ homologous region was amplified by PCR and inserted up stream of the FLEX switch in a plasmid also containing a diphtheria toxin A (DTA) cassette. Next, the 3′ homologous region was amplified by PCR and inserted downstream of the FLEX switch. Independently, the region between the homologies containing the wild-type Satb1 exon 2 was inserted upstream of a neomycin cassette flanked by two frt sites. Next, a third plasmid was generated containing a fusion construct of parts of intron 1 of Satb1 , the sequences encoded in exon 2 including parts of the 5′ UTR and the start codon of Satb1 , the eGFP open reading frame without its start codon and the 3′ UTR of Satb1 . Subsequently, the three plasmids were combined to obtain the final pSatb1-FLEX targeting vector. Mutagenesis of the Satb1 targeting construct To prevent Satb1 TALEN-mediated editing of the TALEN-targeting site in the Satb1 targeting construct we introduced three point mutations in each TALEN-binding region in the Satb1 targeting construct using the QuickChange mutagenesis kit (Promega). Oligonucleotide sequences used for mutagenesis are listed in Supplementary Table 6 . Switching of the FLEX cassette in prokaryotic cells E. coli expressing Cre- recombinase were transformed with the pSatb1-FLEX plasmid following standard transformation protocols. Single bacterial colonies were picked, grown overnight at 37 °C and plasmid DNA was isolated following standard small scale DNA isolation protocols. Using three primers, a PCR reaction was performed on these plasmids to test for successful Cre-mediated recombination ( Supplementary Fig. 2a ). The first primer binds at the 5′ end of the pSatb1-FLEX construct upstream of the first pair of lox sites. The second primer binds at the 3′ end of the pSatb1-FLEX construct downstream of the second pair of lox sites. The third primer binds in the non-switched state upstream of the second primer and results in a 1.8 kb PCR product. After successful recombination this primer is oriented towards the first primer yielding a 1.4 kb PCR product. Oligonucleotide sequences used for the PCR are listed in Supplementary Table 7 . Switching of the FLEX cassette in eukaryotic cells For assessment of Cre-mediated switching, the FLEX cassette from the conditional targeting construct for the murine Satb1 locus (pSATB1-flex) was inserted into the pTriEx-4 Neo Vector (Novagen) harbouring an eukaryotic promoter and thus allowing for eGFP expression after Cre-mediated recombination. Next, NIH3T3 as well as HEK293T cells were seeded in six-well-plate with 6 × 10 5 cells. After ~24 h incubation, cells were transfected with either pTriExSATB1-flex alone or together with a Cre- recombinase encoding plasmid (pCrePac). Cells were transfected using Turbofect (Fermentas). For six-well plates we used 4 μg of each plasmid per well. All transfection experiments were performed according to the manufacturer’s recommended protocol. After 24 h cells were harvested and eGFP expression was determined by flow cytometry. Transfection and cell culture of ES cells JM8A3 murine embryonic stem cells (EuMMCR) were cultured on mitomycin C-inactivated mouse embryonic fibroblast feeder layers with standard murine ES-cell culture conditions. ES cells (1 × 10 7 ) were transfected with the targeting donor plasmid alone or together with TALEN plasmids by electroporation and subsequently seeded on four 10 cm dishes coated with mitomycin C-inactivated mouse embryonic fibroblasts. On day 2 after electroporation selection was initiated by addition of G418 (150 μg ml −1 ) to the culture medium. After G418 selection for 7–9 days individual clones were picked, cultured for 3 more days and genotyped by PCR analysis. Southern blotting Liver genomic DNA (20 μg) of the F1 founder mouse was digested with 50 U Spe I or Eco RV (NEB) respectively in 50 μl overnight at 37 °C. The genomic DNA fragments were separated overnight at 30 V on a 0.7% agarose gel in 1 × TAE buffer containing 1 μg ml −1 ethidium bromide. For depurination, the gel was incubated in 0.25 M HCl for 8 min and washed shortly. The gel was subsequently denatured by incubating two times for 15 min in 0.5 M NaOH/1.5 M NaCl. Next, the gel was neutralized two times for 15 min with 0.5 M Tris (pH 7.5)/1.5 M NaCl. After blotting overnight on a Hybond N+ membrane (GE Healthcare), the nylon membrane was dried at room temperature. The dried membrane was UV-crosslinked by irradiation with 70,000 μJ cm −2 . Next, 10 ml of hybridization buffer (QuikHyb Rapid Hybridization Solution, Agilent) were added and the membrane was incubated for 45 min at 68 °C. Probe (150 ng) was radioactively labelled using random-primer labelling (GE Healthcare) by adding 7 μl radioactively labelled 32 P-dCTP (10 μCi μl −1 ) and purified on a Sephadex-G50 column. The denatured radioactively labelled probe was added to the membrane and incubated for 90 min at 68 °C. Afterwards, the membrane was washed in SDS-containing solutions of SSC with decreasing concentrations of SSC for each washing step. The signal was visualized by incubating the membrane on an X-ray film in the dark for 48 h. X-ray films were developed in a Curix60 developer and digitally scanned. Recombination of the FLEX cassette in murine cells To test the functionality of the targeted allele and the FLEX switch in primary splenocytes and thymocytes, freshly prepared splenic cells and thymocytes were washed in PBS and resuspended in TAT-Cre-containing medium [38] . TAT-Cre protein was added to the culture medium and sterilized by filtration. Cells (1 × 10 6 ) were resuspended in 1 ml of TAT-Cre-containing medium and plated in a well of a 24-well plate for 90 min. After transduction cells were harvested, washed in PBS, resuspended in normal T-cell medium (RPMI containing 10% FCS, 1 mM sodium pyruvate, 2 mM L -glutamine, 1 × nonessential amino acids, 0.1 mM β-mercaptoethanol, 1% pen/strep) and plated in a well of a 24-well plate. After incubation for 16 h, cells were stained with fluorochrome-conjugated monoclonal antibodies at a dilution of 1:100. Antibodies against B220-Allophycocyanin-Cy7 (RA3-6B2, 103224), CD3-Pacific Blue (17A2, 100214), CD4-Peridinin chlorophyll-Cy5.5 (RM4-5, 100540) and CD8-Allophycocyanin (53-6.7, 100712, all from Biolegend) were used. Flow cytometry eGFP reporter activation was assayed by flow cytometry using a BD LSR II (BD Biosciences). Cells were harvested from their culturing plates at the indicated time points after transfection and resuspended in 200 μl of PBS for flow cytometric analysis. Flow cytometry data were analysed using FlowJo VX (Tree Star). At least 25,000 events were analysed for each transfection sample. Statistical analysis Student’s t -tests were performed with SPSS 21.0 software to test for statistical significance of GFP expression in the presence of Cre-recombinase in HEK293T cells. How to cite this article: Sommer, D. et al . Efficient genome engineering by targeted homologous recombination in mouse embryos using transcription activator-like effector nucleases. Nat. Commun. 5:3045 doi: 10.1038/ncomms4045 (2014).